Broad temperature plateau for thermoelectric figure of merit ZT>2 in phase-separated PbTe0.7S0.3 Thermoelectrics interconvert heat to electricity and are of great interest in waste heat recovery, solid-state cooling and so on. The efficiency of thermoelectric materials depends directly on the average ZT (dimensionless figure of merit) over a certain temperature range, which historically has been challenging to increase. Here we report that 2.5% K-doped PbTe 0.7 S 0.3 achieves a ZT of >2 for a very wide temperature range from 673 to 923 K and has a record high average ZT of 1.56 (corresponding to a theoretical energy conversion efficiency of ~20.7% at the temperature gradient from 300 to 900 K). The PbTe 0.7 S 0.3 composition shows spinodal decomposition with large PbTe-rich and PbS-rich regions where each region exhibits dissimilar types of nanostructures. Such high average ZT is obtained by synergistically optimized electrical- and thermal-transport properties via carrier concentration tuning, band structure engineering and hierarchical architecturing, and highlights a realistic prospect of wide applications of thermoelectrics. Raising the efficiency of energy conversion in thermoelectric materials greatly enhances their prospects for extensive commercial applications [1] , [2] . The efficiency of thermoelectric materials is governed by the dimensionless figure of merit, ZT=( α 2 σ / κ ) T , where α , σ , κ and T are the Seebeck coefficient, electrical conductivity, thermal conductivity and absolute working temperature, respectively. In practical applications, the efficiency of a thermoelectric device depends on the material’s average ZT over the entire working temperature range, rather than its maximum ZT. Therefore, it is imperative to raise the average ZT over the whole temperature range of interest [3] . Persistent efforts have been devoted to enhance ZT through increasing the electrical transport ( α and σ ) via carrier concentration tuning [4] , [5] , [6] , [7] and/or band structure engineering (for example, resonant states [8] and band convergence [4] , [5] , [6] , [9] ), and also through lowering the thermal transport ( κ ) by hierarchical architecturing (atomic/nano/mesostructures) [10] , [11] , [12] , [13] . 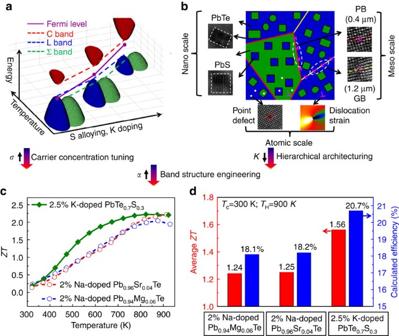Figure 1: High average ZT via synergistically optimized electrical- and thermal-transport properties. (a) A three-dimensional schematic showing the energy difference between conduction (C) band and valence (lightLand heavyΣ) bands as a function of S alloying, K doping and temperature in PbTe. (b) A schematic illustration showing the hierarchical architecture of 2.5% K-doped PbTe0.7S0.3system. The wide colored downward arrows mean that the three aspects collectively contribute to enhance the (average) ZT. (c) ZT and (d) average ZT and calculated efficiency comparisons between 2.5% K-doped PbTe0.7S0.3and other recent reported PbTe-based thermoelectric systems (2.0% Na-doped Pb0.96Sr0.04Te10and 2.0% Na-doped Pb0.94Mg0.06Te11) with high peak ZT values. For convenience, we summarized the Pb Q ( Q =Te, Se, S)-based thermoelectric systems with outstanding ZT values achieved via the above methods in recent years in Supplementary Table 1 . The maximum ZT of the previous materials is high, for example, ZT max >2 of 2.0% Na-doped Pb 0.96 Sr 0.04 Te 10 and 2.0% Na-doped Pb 0.94 Mg 0.06 Te 11 , but the temperature plateau is relatively narrow. In contrast, in the present K-doped PbTe 0.7 S 0.3 system ZT crosses 2 at relatively low temperature of 673 K and remains above 2 until 923 K. This is a wide temperature range known for any material and results in the highest average ZT known (detailed later). For the Pb Q materials, Na and K were generally selected as p-type dopants, not only for tuning the carrier concentration, but also for adjusting the band structure and microstructure, and thus potential for achieving a high ZT. Pei et al. [14] reported that high-performance PbTe can be realized by Na doping through moving the Fermi level into the heavy valence band. Zhang et al. [15] found that heavy K doping in PbTe–PbSe systems could strongly enhance α by activating the heavy-hole band contribution and reduce κ by point defects scattering. In addition, our previous studies indicated that the introduction of Na/K beyond the solubility limit can also result in slightly reduced κ owing to precipitated nanoscale Na/K-rich phases as phonon-scattering sources [16] , [17] . Interestingly, Na doping also can make special shape-control nanostructures [18] . The example of high performance, which involves nanostructuring and heavy valence band engineering, was realized in the Na-doped PbTe–PbS system but not mesostructuring [19] . However, in this case, the bipolar effect degraded α and raised κ at high temperature due to thermal excitation of minority carriers. Compared with Na + (0.97 Å), K + (1.33 Å) can be expected to result in a higher carrier concentration because it is much more similar to Pb 2+ (1.20 Å). In that case the detrimental effect of intrinsic conduction at elevated temperature, that is, bipolar conductivity, is anticipated to be suppressed via increasing the majority carrier (hole) concentration [20] . For microstructures, the density of nanoscaled precipitates could be enhanced through heavy K doping and mesostructuring. Herein, we report that a high thermoelectric ZT max ~2.2 at 923 K can be achieved in the PbTe 0.7 S 0.3 system by optimizing the doping concentration of K. The result in 2.5% K-doped PbTe 0.7 S 0.3 is that the ZT exceeds 2 already at 673 K and remains above it reaching 2.2 at 923 K, creating the broadest temperature range so far in which ZT is above 2. The resulted high ZT average ~1.56 predicts a calculated efficiency of ~20.7% for a temperature drop from 900 to 300 K. Synergistic strategies to enhance ZT The premier role of K doping is to monovalently substitute Pb in PbTe/PbS, which increases the hole concentration and enhances the electrical conductivity σ . By increasing the carrier concentration via K doping, the Fermi energy level is lowered away from the conduction band thereby mitigating the bipolar effect. When S is alloyed into PbTe matrix (the solubility can be tuned by the K doping level, see later), the energy gap between conduction and valence bands of PbTe could be enlarged with increasing temperature so as to further suppress the bipolar effect [19] . Moreover, the Seebeck coefficient α can also benefit from the valence band convergence owing to some incorporation of S on the Te sites [9] . Figure 1a gives a three-dimensional schematic illustration for the temperature-dependent band structure evolution by K doping and S alloying, and thus provides a qualitative reasoning for electrical transport enhancement in K-doped PbTe 0.7 S 0.3 systems. Importantly, K doping also strongly influences the density and morphology of nanoscale precipitates in PbTe and PbS regions, specifically, regular-shaped precipitates exhibit widely in 2.5% K-doped PbTe 0.7 S 0.3 . In addition, mesoscale grain boundaries can be introduced via powder processing. Coupled with atomic-scale lattice distortions, nanoscale regular-shaped precipitates and the fact that the PbTe 0.7 S 0.3 composition is phase separated, an intricate and unique hierarchical architecture can be established to effectively scatter phonons of all length scales, as shown schematically in Fig. 1b . Figure 1: High average ZT via synergistically optimized electrical- and thermal-transport properties. ( a ) A three-dimensional schematic showing the energy difference between conduction ( C ) band and valence (light L and heavy Σ ) bands as a function of S alloying, K doping and temperature in PbTe. ( b ) A schematic illustration showing the hierarchical architecture of 2.5% K-doped PbTe 0.7 S 0.3 system. The wide colored downward arrows mean that the three aspects collectively contribute to enhance the (average) ZT. ( c ) ZT and ( d ) average ZT and calculated efficiency comparisons between 2.5% K-doped PbTe 0.7 S 0.3 and other recent reported PbTe-based thermoelectric systems (2.0% Na-doped Pb 0.96 Sr 0.04 Te 10 and 2.0% Na-doped Pb 0.94 Mg 0.06 Te 11 ) with high peak ZT values. Full size image Through concurrent optimization of electrical and thermal transport properties, we can achieve a maximum ZT of ~2.2 at 923 K in 2.5% K-doped PbTe 0.7 S 0.3 ( Fig. 1c ). To better highlight the advantages of this system, we have compared its temperature-dependence ZT with other reported PbTe-based thermoelectric systems with comparable peak ZT (>2) values, that is, 2.0% Na-doped Pb 0.96 Sr 0.04 Te 10 and 2.0% Na-doped Pb 0.94 Mg 0.06 Te 11 , as seen in Fig. 1c . Impressively, the ZT function of this 2.5% K-doped PbTe 0.7 S 0.3 system exhibits a parabolic climb as temperature increases, while the other reported systems exhibit a more linear climb. As a result, the 2.5% K-doped PbTe 0.7 S 0.3 system shows higher ZT values over a much broader temperature range, in particular, 2.5% K-doped PbTe 0.7 S 0.3 maintains ZT above 2 from 673 to 923 K. The average ZT value is ~1.56, in contrast to ~1.24 and ~1.25 for 2.0% Na-doped Pb 0.96 Sr 0.04 Te 10 and 2.0% Na-doped Pb 0.94 Mg 0.06 Te 11 , respectively ( Fig. 1d ). Considering a hot source of 900 K and a temperature difference across 600 K, a record high efficiency of 20.7% in the 2.5% K-doped PbTe 0.7 S 0.3 system is estimated on the basis of the thermoelectric conversion efficiency [21] , compared with the estimated values of 18.1%, 18.2% in 2.0% Na-doped Pb 0.96 Sr 0.04 Te 10 and 2.0% Na-doped Pb 0.94 Mg 0.06 Te 11 individually. The parabolic climbing feature and large average value of ZT in the 2.5% K-doped PbTe 0.7 S 0.3 system largely come from the extremely low thermal conductivity of a broad range of temperatures, see Supplementary Fig. 1 . Such uniquely low κ of our system can be attributed to its three types of microstructural features. First, compared with Pb 0.96 Sr 0.04 Te and Pb 0.94 Mg 0.06 Te systems, it has been reported that the phase-separated PbTe 0.7 S 0.3 exhibits intrinsically lower thermal conductivities due to the strong phonon scattering at the phase boundaries [22] . Second, a more elaborate and unique hierarchical architecture was established in the present system, in which mesoscale grains include PbTe ones (~1.2 μm) and PbS ones (~400 nm) and chemically ordered layers found in 4-nm cubic precipitates, besides atomic-scale defects and nanoscale precipitates as 2.0% Na-doped Pb 0.96 Sr 0.04 Te 10 and 2.0% Na-doped Pb 0.94 Mg 0.06 Te 11 possess. Third, the volume density of regular-shaped (cubic or near-cubic) precipitates in 2.5% K-doped PbTe 0.7 S 0.3 is nearly 10 times larger than those of platelet-like precipitates in 2.0% Na-doped Pb 0.96 Sr 0.04 Te 10 and 2.0% Na-doped Pb 0.94 Mg 0.06 Te 11 , and thus much stronger phonon scattering can be achieved. Thermoelectric transport properties The thermoelectric properties as a function of temperature are illustrated in Fig. 2 for x mol% K-doped PbTe 0.7 S 0.3 with x =0.5, 1.0, 1.5, 2.0, 2.5 and 3.0. In all samples, σ decreases with increasing temperature ( Fig. 2a ), because of the decreasing carrier mobility. As x increases from 0.5 to 2.0, σ increases and saturates at x =2.0. Specifically, the room temperature σ significantly increases from ~424 S cm −1 for x =0.5 to ~1,740 S cm −1 for x =2.0, and then decreases to ~1,393 Scm −1 for x =3.0. The behaviour of σ as x mainly comes from the competition between the enhanced carrier concentration owing to dissolved K as p-type doping and reduced carrier mobility owing to impurity and/or other defects scattering. 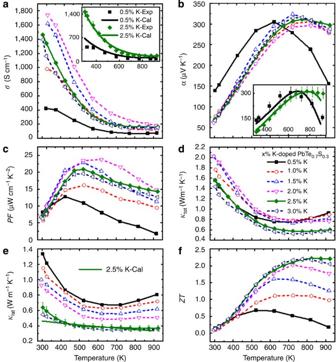Figure 2: Thermoelectric properties as a function of temperature forx% K-doped PbTe0.7S0.3. (a) electrical conductivity, (b) Seebeck coefficient, (c) power factor, (d) total thermal conductivity, (e) lattice thermal conductivity, (f) figure of merit, ZT, the combined uncertainty for all measurements involved in the calculation of ZT is <15% (evaluated in terms of s.d.). Insets inaandbare experimental and calculatedσandαof 0.5% K- and 2.5% K-doped PbTe0.7S0.3. The carrier concentration in the x =0.5 sample was measured as 1.0 × 10 20 cm −3 at 300 K; this value is remarkably enhanced to 2.0 × 10 20 cm −3 in the x =2.5 sample, Supplementary Table 2 . Figure 2: Thermoelectric properties as a function of temperature for x % K-doped PbTe 0.7 S 0.3 . ( a ) electrical conductivity, ( b ) Seebeck coefficient, ( c ) power factor, ( d ) total thermal conductivity, ( e ) lattice thermal conductivity, ( f ) figure of merit, ZT, the combined uncertainty for all measurements involved in the calculation of ZT is <15% (evaluated in terms of s.d.). Insets in a and b are experimental and calculated σ and α of 0.5% K- and 2.5% K-doped PbTe 0.7 S 0.3 . Full size image At relatively low temperatures, the Seebeck coefficient α in Fig. 2b shows an increasing trend, which is typical for a degenerate semiconductor; as the temperature increases further, minority carriers (electrons in this case) arise due to thermal excitation, and the coexistence of majority and minority carriers leads to the so-called bipolar effect, which is believed to be responsible for the saturation of α at elevated temperature. It is also noted that as doping x increases, the saturation temperature of α is pushed to higher temperature ( Fig. 2b ), indicating a suppression of the bipolar effect. The suppression of the bipolar effect can be qualitatively evaluated as follows: the effective band gap ( E g ) can be estimated as E g =2 eT max α max , where α max and T max represents the maximum of α and the temperature at which this value is achieved [4] , E g is enlarged from 0.6 eV at 623 K for x =0.5 to 0.77 eV at 773 K for x =2.5. This suppression effect can be ascribed to the dual function of K doping, that is, carrier concentration tuning and band structure engineering. The increased carrier concentration with a higher K-doping level, Supplementary Table 2 , pulls the Fermi energy level down and away from the conduction band, making the thermal excitation of electrons from valence bands to the conduction band less likely. The introduction of K into the pseudo-binary PbTe–PbS can also adjust the solubility of S in PbTe matrix (discussed later), and thus assist S alloying to tailor a more favourable band structure, that is, moving the conduction and valence bands away from one another in energy, while bringing the light L and heavy Σ valence bands closer [21] . This is similar to the PbTe–MgTe 10 , and PbSe–CdS systems [12] , enhancing α due to the contribution of the heavy valence Σ band. To quantitatively understand the role of K doping and S alloying on the aforementioned carrier concentration tuning and band structure engineering, we performed theoretical calculations on the electrical transport properties of 0.5% K and 2.5% K-doped PbTe 0.7 S 0.3 , based on a three-band ( L+Σ+C ) model and multiple scattering mechanisms (acoustic phonon scattering, point defects scattering and precipitates scattering) [9] , [23] . The details of the calculations can be found in the Supplementary Information. The calculated σ and α in both cases are found to match the experimental results fairly well, shown as the insets in Fig. 2a,b , respectively. Compared with 0.5% K-doped PbTe 0.7 S 0.3 , the heavily K-doped sample 2.5% K-doped PbTe 0.7 S 0.3 possesses a much higher carrier concentration, the energy gap between the conduction band and Fermi level is then enlarged. This means that at the same temperature the bipolar effect can be further suppressed, leaving space for α to climb to a higher level due to the valence band convergence at elevated temperatures ( Figs 1a and 2b ). Collectively, the power factor α 2 σ is remarkably enhanced with a higher K-doping level, which can be attributed to a synergetic effect of carrier concentration promotion, bipolar effect suppression and valence band convergence. Specifically, the peak α 2 σ is raised from ~12.8 μW cm −1 K −2 around 423 K in x =0.5 to ~20.9 μW cm −1 K −2 at 523 K in x =2.5, as shown in Fig. 2d . The contrast is much sharper at 923 K, the α 2 σ increases from ~1.8 μW cm −1 K −2 in x =0.5 to ~14.3 μW cm −1 K −2 in x =2.5, thanks to shifting of α peak to a higher temperature owing to bipolar effect suppression. The total thermal conductivity ( κ tot ) consists of κ ele (electronic thermal conductivity) and κ lat (lattice thermal conductivity). Heat capacity, thermal diffusivity, Lorenz number and electronic thermal conductivity for x% K-doped PbTe 0.7 S 0.3 are shown in Supplementary Fig. 2 . The κ tot in x % K-doped PbTe 0.7 S 0.3 ( x ≤2.0) shows an obvious upturn as temperature goes up, while a flatten trend is observed when x exceeds 2.0 ( Fig. 2d ). The κ lat resembles the trend of κ tot as shown in Fig. 2e . The slight upturns in both κ tot and κ lat again evidence the bipolar effect as mentioned above, and its effect was well suppressed as x was increased over 2.0. With increasing x , κ tot first increases owing to the improved σ , and when x exceeds 2.0, κ tot starts to drop markedly due to precipitated nanoscale phases and other defects ( Fig. 2d ). The effect of K doping on phonon transport can be seen much more clearly through κ lat , which shows a decreasing trend with increasing x ( Fig. 2e ). At room temperature, κ lat decreases from ~1.33 Wm −1 K −1 for x =0.5 to ~0.64 Wm −1 K −1 for x =2.5, and even to ~0.54 Wm −1 K −1 for the x =3.0; correspondingly, κ lat decreases from ~0.81 Wm −1 K −1 to ~0.37 Wm −1 K −1 , and even to ~0.35 Wm −1 K −1 at 923 K. These κ lat are approximately equal to the ‘minimal κ lat ’ value of ~0.36 Wm −1 K −1 for bulk PbTe as calculated by Cahill et al. [24] , and believed to be among the lowest ones reported so far. This reduction in κ lat is significant, which is associated with strong phonon scattering through all-scale hierarchical architectures [3] , [10] , [12] . Combining the ultralow κ , improved σ and enhanced α , a maximum ZT value of ~2.2 at 923 K can be eventually achieved in the 2.5% K-doped PbTe 0.7 S 0.3 sample, as shown in Fig. 2f ; this is among the highest ZT value in the PbTe system reported up to now in bulk thermoelectric materials [10] , [25] . Mesoscale and nanoscale structures To explore the underlying physical mechanisms of the observed low lattice thermal conductivities, we need to look through the microstructural evolution of the x % K-doped PbTe 0.7 S 0.3 systems, especially with the K doping level. Our previous work showed that PbTe 0.7 S 0.3 phase separates (often referred to as spinodal decomposition) into PbTe and PbS phases [22] , and Supplementary Fig. 3 also shows the coexistence of PbTe and PbS phases. Through powder processing, mesoscale PbTe grains (1.2 μm on average, 0.7–1.9 μm in size) and PbS grains (400 nm on average, in the range of 100–800 nm) are produced in all samples ( Fig. 3a,b ; Supplementary Fig. 4 ). Energy dispersive X-ray spectroscopy line scanning and mapping ( Supplementary Fig. 5 ) were utilized to further confirm the separation of PbTe/PbS phases. 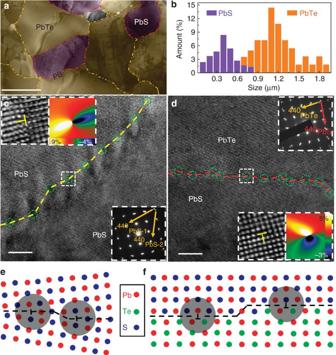Figure 3: Microstructures for mesoscale grains and grain/phase boundaries. (a) Low-magnification TEM image reveals grains and separated phases. Scale bars, 1 μm; (b) grain/phase size distribution histogram; (c,d) lattice images for PbS/PbS grain boundary and PbTe/PbS phase boundary, marked with a yellow and red dashed line, respectively. Edge dislocations along the boundaries are marked with green dashed circles. The electron diffraction pattern, enlarged dislocations and their GPA analysis images are inserted. Scale bars, 5 nm; (e,f) schematics indicating grain and phase boundaries, respectively. Figure 3: Microstructures for mesoscale grains and grain/phase boundaries. ( a ) Low-magnification TEM image reveals grains and separated phases. Scale bars, 1 μm; ( b ) grain/phase size distribution histogram; ( c , d ) lattice images for PbS/PbS grain boundary and PbTe/PbS phase boundary, marked with a yellow and red dashed line, respectively. Edge dislocations along the boundaries are marked with green dashed circles. The electron diffraction pattern, enlarged dislocations and their GPA analysis images are inserted. Scale bars, 5 nm; ( e , f ) schematics indicating grain and phase boundaries, respectively. Full size image High-resolution transmission electron microscopy (HRTEM) was adopted to study the detailed microstructure features on grain/phase boundaries. Figure 3c is a HRTEM image of the PbS/PbS grain boundary (marked with a yellow dashed line) along [001] zone axis, the inserted electron diffraction (ED) pattern indicates its small-angle (~3.4°) feature. An array of edge dislocations marked with green dashed circles can be seen on the grain boundary (tilt grain boundary in this case) between two slightly misaligned grains. The enlarged original and fourier-transformed images of the same dislocation core (marked with a bright dashed square) are inserted in Fig. 3c ; Supplementary Fig. 6b . To investigate the strain variation around the dislocation cores, the high-quality HRTEM image was analysed through geometric phase analysis [26] , [27] . The profile of the strain map of the dislocation core is also inserted in Fig. 3c . The TEM observations also reveal the presence of misfit dislocations and incompletely relaxed strains at the PbTe/PbS phase boundaries, marked with a red dashed line in Fig. 3d , because of the large lattice mismatch (about 6%) between PbTe and PbS [19] . The ED pattern at the phase boundary (inset in Fig. 3d ) reflects the lattice alignment between PbTe and PbS regions. Figure 3e,f are schematic figures showing the dislocations and strain on the PbS/PbS grain boundary and PbTe/PbS phase boundary. Edge dislocations at grain boundary are formed to relieve the strain between misaligned grains and thus their extra semi-atomic planes are along the boundary. On the contrary, edge dislocations at phase boundary are formed to offset the lattice mismatch between two distinct phases and thus their extra semi-atomic planes are perpendicular to the boundary. Despite the difference between the two types of boundaries, they both help scatter long-wavelength phonons. Meanwhile, the atomic-scale distortions at the grain/phase boundaries can act as effective scattering centers for short-wavelength phonons. Besides mesoscale grains, nanoscale precipitates are also found distributed widely but distinctly in the PbTe and PbS regions for all samples. This is a unique phase separation feature in the PbTe 0.7 S 0.3 composition that is not found in other nanostructured PbTe-based systems, which typically have a main PbTe matrix with small nucleated nanostructures grown inside. It is very interesting to find that in each of the PbTe and PbS regions of PbTe 0.7 S 0.3 the density and morphology of these nanoscale precipitates can be tuned by the K doping level. Two sets of figures showing the evolution of precipitates in PbS and PbTe regions with the K doping level are shown in Fig. 4a–d ; Supplementary Fig. 7 , respectively. 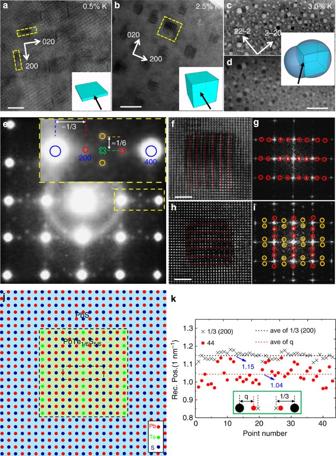Figure 4: Microstructures for nanoscale precipitates. (a,b) Lattice images of 0.5% K- and 2.5% K-doped PbTe0.7S0.3depicting platelet-like precipitates and cubic precipitates, respectively. Scale bars, 5 nm (a); 10 nm (b); (c,d) BF-TEM and HAADF images of 3.0% K-doped PbTe0.7S0.3depicting multiple-sphere precipitates; three-dimensional schematic figures for platelet-like, cubic and multiple-sphere precipitates are inserted, separately, the arrowheads indicate the directions of the TEM observations. Scale bars, 50 nm. (e) Electron diffraction pattern ofb, near-1/3 (2 0 0), near-(1 1/3 0) superlattices and a kinematically forbidden (1 0 0) reflection spot are marked with red, yellow circles and a green cross. (f,h) Enlarged images of cubic precipitates; the three-layered structure is reflected with red dashed lines. Scale bars, 2 nm. (g,i) Fast fourier-transformed images offandhsuperlattices are marked. (j) The atomic model of cubic precipitates, the dashed rectangle indicates the unit cell of superlattice spots. (k) Statistical reciprocal positions of near-1/3 (2 0 0) superlattice spots (red dots) and the 1/3 (2 0 0) (black crosses, non-existed) are counted. Their average values are also shown. Figure 4: Microstructures for nanoscale precipitates. ( a , b ) Lattice images of 0.5% K- and 2.5% K-doped PbTe 0.7 S 0.3 depicting platelet-like precipitates and cubic precipitates, respectively. Scale bars, 5 nm ( a ); 10 nm ( b ); ( c , d ) BF-TEM and HAADF images of 3.0% K-doped PbTe 0.7 S 0.3 depicting multiple-sphere precipitates; three-dimensional schematic figures for platelet-like, cubic and multiple-sphere precipitates are inserted, separately, the arrowheads indicate the directions of the TEM observations. Scale bars, 50 nm. ( e ) Electron diffraction pattern of b , near-1/3 (2 0 0), near-(1 1/3 0) superlattices and a kinematically forbidden (1 0 0) reflection spot are marked with red, yellow circles and a green cross. ( f , h ) Enlarged images of cubic precipitates; the three-layered structure is reflected with red dashed lines. Scale bars, 2 nm. ( g , i ) Fast fourier-transformed images of f and h superlattices are marked. ( j ) The atomic model of cubic precipitates, the dashed rectangle indicates the unit cell of superlattice spots. ( k ) Statistical reciprocal positions of near-1/3 (2 0 0) superlattice spots (red dots) and the 1/3 (2 0 0) (black crosses, non-existed) are counted. Their average values are also shown. Full size image We first consider the PbTe regions. Supplementary Fig. 7a is a lattice image for PbTe-rich region of the x =0.5 sample showing roughly homogeneous contrast, with only some weak-contrast particles about one atom layer in size. This is an indication of a possible pseudo-solid solution (point defect) [27] . When x increases to 2.0, slightly small precipitates with a grown size (around 2 nm) can be seen ( Supplementary Fig. 7b ). A further increase of x to 2.5 results in a high density of precipitates (around 5 nm, 1–12 nm in size, Supplementary Fig. 8c ) overspreading ( Supplementary Fig. 7c ). The morphology of these precipitates is close to cubic. The fast fourier-transformed image of Supplementary Fig. 7c shows slight peak splitting of high-order reflection spots, for example, (400) spots ( Supplementary Fig. 7d ) based on which, the composition of precipitates can be estimated as PbTe 0.75 S 0.25 (the exact composition of K is difficult to detect) [11] , [16] , [17] . Then we need to look through the evolution of precipitates in PbS regions with the K doping level, as shown in Fig. 4a–d . When PbTe 0.7 S 0.3 is slightly doped ( x =0.5), platelet-like precipitates [11] , [16] , [17] can be seen along the [001] zone axis ( Fig. 4a ). The platelet-like precipitates are found to be in (100) or (010) planes with a width of around 4 nm and a thickness of about 1–2 atomic layers ( Supplementary Fig. 8a ). As x increases to 2.5, cubic precipitates with all edges along <100> directions are detected with an average size of 4 nm (varying from 1–7 nm) ( Fig. 4b ; Supplementary Figs 8b and 9a,b ). The low-magnification bright-field TEM (BF-TEM) and high-angle annular dark field (HAADF) images show a consistently high density of cubic precipitates distributed in the whole area ( Supplementary Fig. 9a,b ). The cubic precipitates show darker contrast in BF-TEM images while brighter contrast in HAADF images, indicating that they are PbTe rich embedded in a PbS-rich matrix. Interestingly, some precipitates in the PbS-rich matrix form as binary pairs of cubic precipitates ( Supplementary Fig. 9a,b ) with opposite contrast. The additional parts of the binary cubic precipitates exhibit darker contrast in the HAADF image (brighter contrast in the BF-TEM image) than the matrix hints that they are K-rich. These peculiar precipitates, few but regular (cubic) in the x =2.5 sample, are more numerous but irregular (spherical) in the x =3.0 sample, as shown in Fig. 4c,d ; Supplementary Fig. 9c,d . These special morphologies of the x =3.0 sample can be called as multiple-sphere ones, the K-rich spheres seem stuck to PbTe-rich ones. Three parts of the multiple-sphere precipitates exhibit endotaxial relationship with little lattice parameter difference, as shown in Supplementary Fig. 10 . It is seen that the multiple-sphere precipitates of the x =3.0 sample possess higher density of interfaces than the cubic ones of the x =2.5 sample, that is, stronger phonon scattering, and thus contributes to lower thermal conductivities, as shown in Fig. 2d,e . Our data clearly show that with the increase of K doping, the number density of precipitates in the PbS regions is almost unchanged, but the morphology changes significantly, from platelet-like for x <2.5 to cubic for x =2.5, and finally to multiple sphere for x >2.5. The three-dimensional schematics, inserted in Fig. 4a–d , show the corresponding morphology of platelet-like, cubic and multiple-sphere ones, respectively, and the arrowheads indicate the directions of the TEM observations. The cubic precipitates can be regarded as grown from the platelets along the normal direction of the plane, while the multiple-sphere precipitates can be imagined as {100} swollen cubic ones. Here, it is necessary to provide a detailed structural analysis for the cubic precipitates in PbS regions of the 2.5% K-doped PbTe 0.7 S 0.3 sample, which exhibits the highest thermoelectric performance. Figure 4e represents a [001] zone axis ED pattern of Fig. 4b , showing obvious superlattice spots besides the fundamental Bragg peaks from the matrix. Two sets of superlattice spots marked with red circles betray modulation wave vectors of 1/3(2, 0, 0) and 1/3(0, 2, 0) [22] , [28] , while another two sets of superlattice spots marked with yellow circles are from the modulations of the kinematically forbidden reflections spots ( h 00) and (0 k 0) (marked with green cross, h and k are odd). These four sets of superlattice spots are actually from different precipitates, and two of such precipitates are shown in Fig. 4f,h . Three-layered lattices can be found in both ( Fig. 4f,h ), which are consistent with one set of 1/3(2, 0, 0) superlattice spots ( Fig. 4g ) and two sets of 1/3(0, 2, 0) and (1, 1/3, 0) ones ( Fig. 4i ). On the basis of the above structural information, the atomic model of cubic precipitates in the PbS regions can be established as shown in Fig. 4j . The layered structure can be expressed as one Te atom for every five S atoms (chemical ordering), roughly predicting the composition of precipitates as PbS 5/6 Te 1/6 (refs 22 , 28 , 29 ). Furthermore, the above 1/3 superlattice spots can be expressed more accurately as (1/3- ε )(2, 0, 0) or (1/3- ε )(0, 2, 0), with a deviation parameter ε (refs 22 , 28 ). The existing deviation from the ideal 1/3 position is due to the expanded lattice parameter caused by the substitution of Te on S sites. We did statistics of the distance between both these near-1/3 superlattice spots (red spots) and the 1/3 (200) (black spots) to the center spot and the average ε can be estimated as 0.03 ( Fig. 4k ). The chemical-ordered layers inside 4-nm cubic precipitates are peculiar in the 2.5% K-doped PbTe 0.7 S 0.3 sample, which could act as additional short-wavelength phonon scattering centers, similar with the displacement layers in the PbTe–PbSnS 2 and SnSe system [30] , [31] . We expect that these atomically ordered layers play an important role in the elaborate hierarchical architecture to effectively scatter phonons at particular length scales. It is clearly seen that K doping is important in defining the density and morphology of precipitates in the PbTe/PbS regions. Our previous work reported that the solubility of Na is low in PbTe (~0.5%) while high in PbS (~2.0%) [16] . The situation of K doping in PbTe and PbS is similar, but with comparably lower solubility, which means that the microstructure of PbTe/PbS is more sensitive to K doping than Na doping. Thus, the influence of K in PbTe and PbS regions should be distinct, especially when its concentration is above the solid solubility. For low K doping (for example, x =0.5), K mainly exists in the form of point defects, and thus slightly influences the density or morphology of precipitates. For higher K doping (for example, x =2.5), the excess K causes PbS separation from the PbTe matrix. The reason is that the defect-formation energy of K in PbS-rich precipitates is much lower than that in the PbTe matrix, that is, PbS-rich precipitates can dissolve more K [16] , [18] . Therefore, both the size and density of PbS-rich precipitates in the PbTe regions increase, as the K content increases. By contrast, there is no way for the excess K in the PbS regions to dissolve through separating more PbTe-rich precipitates, since the defect-formation energy of K in PbTe-rich precipitates is much higher. The only choice for the excess K is to segregate at the interfaces between PbTe-rich precipitates and PbS matrix. It is the segregation of K at the {100} precipitate/matrix interfaces that results in cubic morphology for precipitates in x =2.5 sample, which is similar with the morphology control of Na doping in the PbTe–PbS system [18] . By further increasing the concentration of K (for example, x =3.0), these interfaces can no longer withstand the enhanced K segregation, but compel some K to diffuse into the matrix. That is probably the reason why the multiple-sphere precipitates are present in the 3.0% K-doped PbTe 0.7 S 0.3 sample, in which the swollen parts (brighter in BF-TEM image while darker in HAADF image, Fig. 4c,d ) should be K-rich. Structure-thermal conductivity properties correlation To better understand the intrinsic relationship between the hierarchical structure and the low κ lat of 2.5% K-doped PbTe 0.7 S 0.3 , we performed κ lat calculations, based on Callaway’s semi-classical model [32] , with various scattering processes being integrated [27] . The detailed information of the calculations is presented in Supplementary Information. The calculated κ lat for 2.5% K-doped PbTe 0.7 S 0.3 shows good agreement with the experimental one, see Fig. 2e . The model suggests that the phonon scattering by the nanoscale precipitates shall take the major responsibility for the low κ lat , although phonon scatterings by other length-scale sources also contribute. Impressively, the volume density of regular-shaped precipitates of 2.5% K-doped PbTe 0.7 S 0.3 can be estimated as >10 times larger than those of platelet-like precipitates in 2.0% Na-doped Pb 0.96 Sr 0.04 Te 10 and 2.0% Na-doped Pb 0.94 Mg 0.06 Te 11 , although they possess a similar number density (10 23 m −3 ), and thus phonons with mediate mean free paths can be effectively scattered in the present system [33] . Meanwhile, the atomically ordered layers inside the 4-nm cubic precipitates can additionally scatter phonons with short wavelength. Therefore, nanoscale precipitates combined with long-wavelength phonon scattering centers (mesoscale grains), and short-wavelength phonon scattering centers (atomically ordered layers and atomic-scale lattice distortions), define a all-scale hierarchical architecture to scatter phonons. This collective phonon scattering appears more effective than the already remarkable ones observed in 2.0% Na-doped Pb 0.96 Sr 0.04 Te 10 and 2.0% Na-doped Pb 0.94 Mg 0.06 Te 11 , as compared in Fig. 1b . Thus, the lowest thermal conductivities were obtained in 2.5% K-doped PbTe 0.7 S 0.3 among all Pb Q systems, namely, κ la t : 0.64 Wm −1 K −1 at 300 K and 0.37 Wm −1 K −1 at 923 K; κ tot : 1.56 Wm −1 K −1 at 300 K and 0.6 Wm −1 K −1 at 923 K ( Fig. 2e,f ; Supplementary Fig. 1d,e ). The consequence of this is that very high ZT values over a broad range of temperatures (300–900 K) can be achieved. The introduction of K in the phase-separated PbTe 0.7 S 0.3 system causes profound and multiple effects: (a) it enhances the carrier concentration as in traditional p-type doping for high electrical conductivity; (b) it suppresses the bipolar effect by pushing down the Fermi level away from the conduction band and assisting S alloying to tailor a more favourable band structure, so as to enhance the Seebeck coefficients at elevated temperatures; (c) it helps to form abundant nanoscale regular-shaped precipitates, which together with atomic-scale defects and mesoscale grains can effectively scatter phonons on multiple length scales, leading to the lowest lattice thermal conductivities (0.64 Wm −1 K −1 at 300 K and 0.37 Wm −1 K −1 at 923 K) reported in any Pb Q system. The integration of all these effects in 2.5% K-doped PbTe 0.7 S 0.3 not only pushes ZT to ~2.2 at 923 K but also creates the first example of a material with the broadest plateau of ZT>2 from 673 to 923 K. Therefore, the material achieves a record high average ZT of ~1.56 making it unique in being capable of a high theoretical conversion efficiency of ~20.7% in a device implementation. Synthesis A series of x mol% K-doped PbTe 0.7 S 0.3 ( x =0.5, 1.0, 1.5, 2.0, 2.5, 3.0) samples were synthesized following the processes as below: raw materials weighing a total 20 g (Pb, Te, S and K) were melted into ingots at 1,323 K over 10 h inside evacuated fused silica tubes. These tubes were then furnace cooled to room temperature and the obtained ingots were crushed into powders <5 mm 3 and further ground with a mortar and pestle. After sieving only powders smaller than 53 μm 3 were used for next steps. The selected fine powders were densified using spark plasma sintering (SPS, SPS-211Lx, Dr Sinter) at 823 K for 10 min with a 60 MPa uniaxial pressure. Characterization Corresponding σ and α were measured simultaneously from room temperature to about 923 K under the protection of He gas using a ULVAC-RIKO ZEM-3 instrument system. The carrier concentration was derived by the low magnetic field (0 to 1.25 T) Hall coefficient measured with Lakeshore instruments. The κ tot was calculated using the formula κ tot =DC p ρ , where the thermal diffusivity D was measured using the laser flash method in a commercial Netzsch LFA-457 instrument from 300 to 923 K, and the specific heat capacity C p was derived from a reference sample (Pyroceram 9606), ρ is the sample density, which was measured using a gas pycnometer (Micromeritics AccuPyc 1340). The TEM specimens were prepared by conventional standard methods, that is, cutting, grinding, dimpling, polishing and Ar-ion milling with a liquid nitrogen cooling stage. S/TEM investigations were carried out in a JEOL 2100F microscope. How to cite this article: Wu, H. J. et al. Broad temperature plateau for thermoelectric figure of merit ZT>2 in phase-separated PbTe 0.7 S 0.3 . Nat. Commun. 5:4515 doi: 10.1038/ncomms5515 (2014).